Localized light-induced protein dimerization in living cells using a photocaged dimerizer Regulated protein localization is critical for many cellular processes. Several techniques have been developed for experimental control over protein localization, including chemically induced and light-induced dimerization, which both provide temporal control. Light-induced dimerization offers the distinct advantage of spatial precision within subcellular length scales. A number of elegant systems have been reported that utilize natural light-sensitive proteins to induce dimerization via direct protein–protein binding interactions, but the application of these systems at cellular locations beyond the plasma membrane has been limited. Here we present a new technique to rapidly and reversibly control protein localization in living cells with subcellular spatial resolution using a cell-permeable, photoactivatable chemical inducer of dimerization. We demonstrate light-induced recruitment of a cytosolic protein to individual centromeres, kinetochores, mitochondria and centrosomes in human cells, indicating that our system is widely applicable to many cellular locations. Vital cellular processes, such as signalling, migration, growth and division, require the participation of tens to hundreds of different proteins whose localization and interactions are dynamically regulated in space and time. Experimentally controlling protein localization is a powerful approach for investigating these complex systems. Light-induced protein dimerization can provide both temporal and spatial precision for such manipulations [1] . Similar to the more mature technique of chemically induced dimerization [2] , [3] , [4] , light-induced dimerization exploits a pair of specialized protein domains that can be driven into a high-affinity binding state by an experimental stimulus, such as the addition of a small molecule or illumination with a specific wavelength of light. These dimerization domains are genetically fused to two proteins of interest, which allows for experimental control over their interaction. The state-of-the-art for light-induced protein dimerization techniques utilize either photosensitive proteins [5] , [6] , [7] , [8] or a photocaged chemical dimerizer, rapamycin [9] , [10] , and each technique offers a different set of strengths and weaknesses. Inducing dimerization with subcellular spatial control requires that the photoactivated component remain persistently localized at the site of activation. The reported forms of photocaged rapamycin release diffusible, free rapamycin upon uncaging and therefore have limited potential for spatially controlled dimerization [3] . In principle, a photosensitive protein can be stably targeted to any location in the cell by genetic fusion to an appropriate anchoring domain. In practice, the photosensitive protein systems all function at the plasma membrane, and some have been used to regulate transcription [5] , [6] , [7] , but application of most of these systems to a variety of intracellular locations has not been reported. Only one system [5] has been tested with a diverse set of anchoring domains, and in that study approximately half of the fusion proteins tested localized properly [11] . Here we report a light-induced dimerization system that is broadly applicable at a variety of locations in human cells. This system utilizes a modular dimerizer consisting of a photocaged ligand joined by a flexible linker to a different, non-caged ligand. The two orthogonal ligands allow specific, high-affinity binding to their cognate receptors and, therefore, heterodimerization of proteins of interest fused to the receptors. We demonstrate light-induced recruitment of a cytosolic reporter protein to centromeres, kinetochores, centrosomes and mitochondria in living human cells using this novel cell-permeable photocaged chemical dimerizer. Molecular design of the photocaged dimerizer To function successfully, a photocaged chemical dimerizer should enter living cells, stably bind the receptor for the non-caged ligand and bind the receptor for the photocaged ligand only after uncaging ( Fig. 1 ). To ensure that the dimerizer remains stably bound to the receptor for the uncaged ligand, we employed a selective, covalent labelling system. This approach allows saturation of the first receptor with the caged dimerizer followed by washout of any free dimerizer, which would otherwise nonproductively compete for binding the second receptor after uncaging. For our non-caged covalent ligand/receptor pair, we chose the Halotag system, which consists of a bacterial alkyldehalogenase enzyme mutated to irreversibly form a covalent bond with chloroalkyl-containing substrates [12] . This system offers rapid covalent protein labelling that is bioorthogonal in human cells, and it has been successfully utilized for protein heterodimerization [13] , [14] . For clarity, we will refer to the Halotag protein as Haloenzyme and the chlorohexane group as Haloligand. 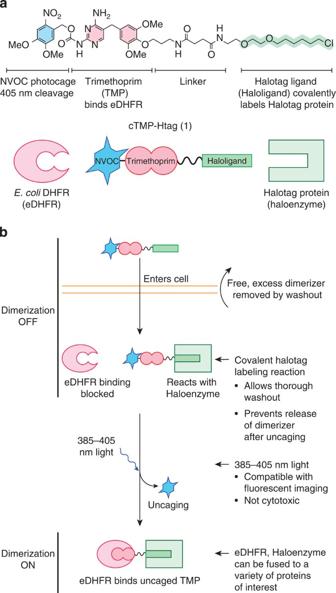Figure 1: Design of photocaged dimerizer cTMP-Htag. (a) Chemical structure and schematic diagrams of cTMP-Htag1and its two receptors:E. coliDHFR (eDHFR) and the Halotag protein (Haloenzyme). (b) Schematic of light-induced protein dimerization in living cells via cTMP-Htag. The cell-permeable photocaged dimerizer enters cells and irreversibly reacts with the Haloenzyme. Any unreacted dimerizer is removed by washout. The photocage prevents binding with eDHFR before illumination, and is removed by irradiation with ~385–405 nm light, allowing eDHFR to bind the uncaged TMP group, thus dimerizing eDHFR and Haloenzyme. Figure 1: Design of photocaged dimerizer cTMP-Htag. ( a ) Chemical structure and schematic diagrams of cTMP-Htag 1 and its two receptors: E. coli DHFR (eDHFR) and the Halotag protein (Haloenzyme). ( b ) Schematic of light-induced protein dimerization in living cells via cTMP-Htag. The cell-permeable photocaged dimerizer enters cells and irreversibly reacts with the Haloenzyme. Any unreacted dimerizer is removed by washout. The photocage prevents binding with eDHFR before illumination, and is removed by irradiation with ~385–405 nm light, allowing eDHFR to bind the uncaged TMP group, thus dimerizing eDHFR and Haloenzyme. Full size image For the photocaged ligand, we chose trimethoprim (TMP), a dihydrofolate reductase (DHFR) inhibitor, which is selective for bacterial versus mammalian forms of DHFR [15] . The combination of TMP and Escherichia coli DHFR (eDHFR) has been well validated as a bioorthogonal ligand/receptor pair in eukaryotic cells [16] , [17] , [18] , [19] , [20] . TMP is small and structurally simple but also amenable to synthetic derivatization. Linkers can be added to the para position of the trimethoxyphenyl ring of TMP without interfering with DHFR binding [16] . By contrast, the 2,4-diaminopyrimidine ring of TMP is buried in the DHFR substrate pocket [21] , so we predicted that adding a bulky photocage to this group would effectively block DHFR binding. Neither photocaged TMP nor a photocaged modular chemical inducer of dimerization have been reported. Haloenzyme and eDHFR are globular proteins of 294 and 158 amino acids, respectively, comparable to GFP (239 amino acids). Like GFP, both have been successfully fused to the amino (N) and carboxy (C) termini of a variety of proteins [12] , [18] , [19] , [22] . The diaminopyrimidine ring of TMP was caged as the 6-nitroveratryl carbamate (NVOC) [23] . Exocyclic amines analogous to those of TMP have been photocaged using carbamate linkages [24] , which rapidly decarboxylate upon photocleavage, releasing the native amine [23] , [25] . Combining photocaged TMP with the Haloligand yielded cTMP-Htag ( 1 , Fig. 1a ). We also synthesized and tested the non-photocaged analogue TMP-Htag ( 2 , Fig. 2 ). For synthetic scheme and characterization details, see Supplementary Figs 1–15 and Supplementary Methods . NVOC can be released with light at 365–420 nm, which is not acutely cytotoxic [23] , [26] . In addition, the absorption spectrum of NVOC is sufficiently blueshifted to protect it from undesired cleavage at wavelengths commonly used for imaging (for example, 488 nm) ( Fig. 2 ). 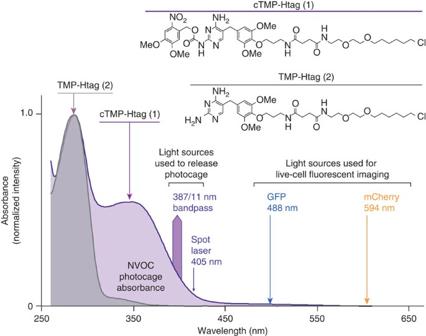Figure 2 Ultraviolet (UV)–visible absorbance spectra of dimerizers. Chemical structures and normalized UV–visible spectra (260–600 nm) of cTMP-Htag (1, in 90% phosphate-buffered saline (PBS) pH 7.4/10% dimethyl sulphoxide) and the non-caged analogue TMP-Htag (2, in 75% PBS pH 7.4/25% DMSO). Light sources used for uncaging (387/11, 405 nm) or for imaging (488, 594 nm) are indicated. Figure 2 Ultraviolet (UV)–visible absorbance spectra of dimerizers. Chemical structures and normalized UV–visible spectra (260–600 nm) of cTMP-Htag ( 1 , in 90% phosphate-buffered saline (PBS) pH 7.4/10% dimethyl sulphoxide) and the non-caged analogue TMP-Htag ( 2 , in 75% PBS pH 7.4/25% DMSO). Light sources used for uncaging (387/11, 405 nm) or for imaging (488, 594 nm) are indicated. Full size image Light-induced protein dimerization in living cells We first tested the ability of cTMP-Htag to recruit a freely diffusible protein to centromeres. Centromeres are specialized chromatin domains that host the dynamically regulated localization of >100 proteins essential for cell division, making them highly attractive targets for light-inducible dimerization [27] . Vital centromere functions that require regulated protein localization include maintenance of sister chromatid cohesion and kinetochore assembly. Light-induced dimerization at centromeres has not been reported using any of the published systems. We constructed a HeLa cell line expressing E. coli DHFR (eDHFR) fused to mCherry (mCherry–eDHFR) and the human centromere protein CENPB fused to GFP and Haloenzyme (CENPB–GFP-Halo). CENPB specifically binds to a short sequence in the repetitive DNA present at all typical human centromeres (except the Y chromosome) [28] , [29] . As expected, CENPB–GFP-Halo localizes to centromeres, and mCherry–eDHFR localizes diffusely in untreated cells. cTMP-Htag enters living cells, and incubation with 20 μM cTMP-Htag for 30 min results in full occupancy of the available Haloenzyme sites in the cell ( Fig. 3 ). Cells treated with cTMP-Htag and exposed to a short pulse of 387 (±6) nm light exhibited dramatic recruitment of mCherry–eDHFR to centromeres with a t 1/2 of ~15 s ( Fig. 4a,b ). No effect was observed in control experiments testing extended exposure to 488 nm light or the absence of cTMP-Htag ( Supplementary Fig. 16 ). Next, we used a targeted 405 nm laser to achieve rapid and spatially defined recruitment to an individual centromere ( Fig. 4c ). 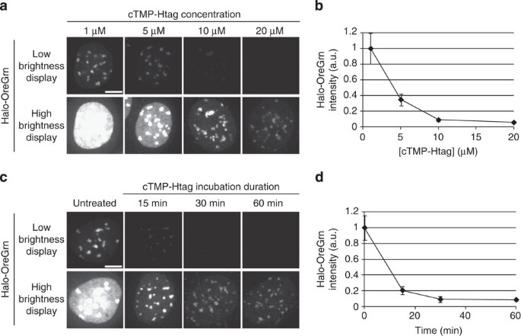Figure 3: cTMP-Htag enters living cells. The extent of cTMP-Htag reaction with CENPB-Haloenzyme as a function of cTMP-Htag concentration or treatment time was measured using a dye-blocking assay. Cells expressing CENPB-Haloenzyme (without GFP) were incubated with cTMP-Htag, washed, treated with 100 nM Halotag-Oregon Green (Halo-OreGrn) for 20 min, then washed again before imaging. Decreased Halo-OreGrn indicates cTMP-Htag occupancy of CENPB-Haloenzyme sites. Each Halo-OreGrn image is displayed at two brightness levels to aid visualization. Within each row, all the images are displayed using identical brightness levels. (a,b) Cells were treated with 1, 5, 10 or 20 mM cTMP-Htag for 1 h, then treated with Halo-OreGrn as described above. Treatment with 10 μM cTMP-Htag for 1 h is sufficient to block ~90% of Halo-OreGrn binding. (c,d) Cells were treated with 20 μM cTMP-Htag for 15, 30 or 60 min, or left untreated as control, then treated with Halo-OreGrn as described above. Treatment with 20 μM cTMP-Htag for 30 min is sufficient to block ~90% of Halo-OreGrn binding. Images (a,c) are maximum-intensity projections of representative cells from each condition. Average Halo-OreGrn intensity at centromeres was quantified for each condition (b,d). Error bars represent s.d. (n≧15 fields for each data point, multiple cells per field). a.u., arbitrary unit. Figure 3: cTMP-Htag enters living cells. The extent of cTMP-Htag reaction with CENPB-Haloenzyme as a function of cTMP-Htag concentration or treatment time was measured using a dye-blocking assay. Cells expressing CENPB-Haloenzyme (without GFP) were incubated with cTMP-Htag, washed, treated with 100 nM Halotag-Oregon Green (Halo-OreGrn) for 20 min, then washed again before imaging. Decreased Halo-OreGrn indicates cTMP-Htag occupancy of CENPB-Haloenzyme sites. Each Halo-OreGrn image is displayed at two brightness levels to aid visualization. Within each row, all the images are displayed using identical brightness levels. ( a , b ) Cells were treated with 1, 5, 10 or 20 mM cTMP-Htag for 1 h, then treated with Halo-OreGrn as described above. Treatment with 10 μM cTMP-Htag for 1 h is sufficient to block ~90% of Halo-OreGrn binding. ( c , d ) Cells were treated with 20 μM cTMP-Htag for 15, 30 or 60 min, or left untreated as control, then treated with Halo-OreGrn as described above. Treatment with 20 μM cTMP-Htag for 30 min is sufficient to block ~90% of Halo-OreGrn binding. Images ( a , c ) are maximum-intensity projections of representative cells from each condition. Average Halo-OreGrn intensity at centromeres was quantified for each condition ( b , d ). Error bars represent s.d. ( n ≧ 15 fields for each data point, multiple cells per field). a.u., arbitrary unit. 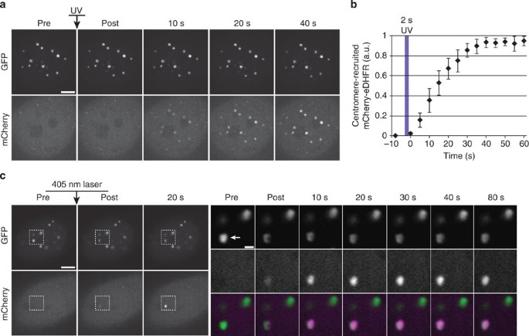Figure 4: Light-induced dimerization at centromeres. Cells expressing CENPB–GFP-Haloenzyme and mCherry–eDHFR were treated with 20 μM cTMP-Htag for 1 h, then washed before imaging. (a) Cell-wide recruitment of mCherry–eDHFR to centromere-localized CENPB–GFP–Haloenzyme in response to a 2-s pulse of 387(±5.5) nm light. (b) Average mCherry–eDHFR centromere intensity at time points before and after uncaging, error bars represent s.d. (n=10 cells). (c) A single centromere (indicated by arrowhead in inset) was irradiated with a 405 nm laser to induce mCherry–eDHFR recruitment. Insets show boxed regions in GFP (top row) and mCherry (middle row) and colour-merge (bottom row) from indicated time points. Scale bars, 5 or 1 μm in insets. a.u., arbitrary unit. Full size image Figure 4: Light-induced dimerization at centromeres. Cells expressing CENPB–GFP-Haloenzyme and mCherry–eDHFR were treated with 20 μM cTMP-Htag for 1 h, then washed before imaging. ( a ) Cell-wide recruitment of mCherry–eDHFR to centromere-localized CENPB–GFP–Haloenzyme in response to a 2-s pulse of 387(±5.5) nm light. ( b ) Average mCherry–eDHFR centromere intensity at time points before and after uncaging, error bars represent s.d. ( n =10 cells). ( c ) A single centromere (indicated by arrowhead in inset) was irradiated with a 405 nm laser to induce mCherry–eDHFR recruitment. Insets show boxed regions in GFP (top row) and mCherry (middle row) and colour-merge (bottom row) from indicated time points. Scale bars, 5 or 1 μm in insets. a.u., arbitrary unit. Full size image Photochemical uncaging is irreversible, but TMP-eDHFR binding is reversible, and there is precedent for using free TMP to compete with a TMP-based chemical dimerizer [19] . Therefore we predicted that addition of free TMP would compete with uncaged TMP-Htag for eDHFR binding, leading to reversal of induced dimerization. Following light-induced recruitment, incubation with excess TMP released mCherry–eDHFR from centromeres within 6 min, demonstrating a full OFF–ON–OFF cycle of experimental control ( Fig. 5a,b ). Furthermore, washout of excess TMP led to relocalization of mCherry–eDHFR to centromeres ( Fig. 5c ). 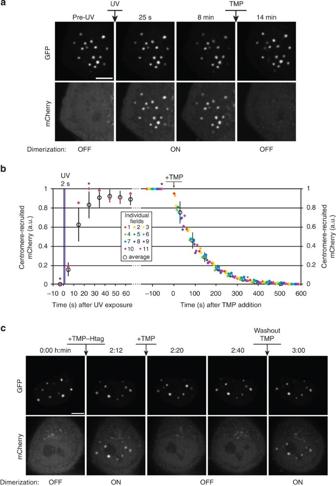Figure 5: Dimerization reversal by addition of free TMP. Cells were expressing CENPB–GFP-Haloenzyme and mCherry–eDHFR. (a,b) Cells were treated with 20 μM cTMP-Htag for 1 h, then washed before imaging. Eleven fields of interphase cells were sequentially activated with a 2 s pulse of ultraviolet (UV) light, then imaged every 10 s for 60 s. Eight minutes after the 11th field was photoactivated, all the fields were imaged again, then TMP was added to a final concentration of 100 μM. Each field was imaged every minute for 10 min. Image acquisition and stage movement took ~4.5 s for each field. Selected images from the 11th field (a). mCherry intensity at centromeres was quantified (b). For the photoactivation phase of the experiment, centromere intensity levels were normalized for each field, then averaged over all the fields for each time point. This average, as well as the normalized values for the 11th field are plotted. For the TMP-addition phase of the experiment, measurements for each field at each time point are plotted. mCherry intensity was normalized for each field, then averaged across all the fields for each 1-min image acquisition cycle. Averages are plotted as a function of the average image acquisition time during each cycle (for instance, ~24 s after the addition of TMP for the first cycle). Measurements of field 11 corresponding to the images displayed inaare marked with an asterisk (*). Error bars represent s.d. (c) Cells were treated with 1 μM TMP-Htag for 30 min, then washed and imaged ~2 h later. TMP was added to a final concentration of 100 μM, resulting in the loss of dimerization within 8 min. TMP was removed by washout, resulting in the recovery of dimerization within 20 min. Scale bars, 5 μm. Figure 5: Dimerization reversal by addition of free TMP. Cells were expressing CENPB–GFP-Haloenzyme and mCherry–eDHFR. ( a , b ) Cells were treated with 20 μM cTMP-Htag for 1 h, then washed before imaging. Eleven fields of interphase cells were sequentially activated with a 2 s pulse of ultraviolet (UV) light, then imaged every 10 s for 60 s. Eight minutes after the 11th field was photoactivated, all the fields were imaged again, then TMP was added to a final concentration of 100 μM. Each field was imaged every minute for 10 min. Image acquisition and stage movement took ~4.5 s for each field. Selected images from the 11th field ( a ). mCherry intensity at centromeres was quantified ( b ). For the photoactivation phase of the experiment, centromere intensity levels were normalized for each field, then averaged over all the fields for each time point. This average, as well as the normalized values for the 11th field are plotted. For the TMP-addition phase of the experiment, measurements for each field at each time point are plotted. mCherry intensity was normalized for each field, then averaged across all the fields for each 1-min image acquisition cycle. Averages are plotted as a function of the average image acquisition time during each cycle (for instance, ~24 s after the addition of TMP for the first cycle). Measurements of field 11 corresponding to the images displayed in a are marked with an asterisk (*). Error bars represent s.d. ( c ) Cells were treated with 1 μM TMP-Htag for 30 min, then washed and imaged ~2 h later. TMP was added to a final concentration of 100 μM, resulting in the loss of dimerization within 8 min. TMP was removed by washout, resulting in the recovery of dimerization within 20 min. Scale bars, 5 μm. Full size image To test the general applicability of our system, we constructed Haloenzyme–GFP fusion proteins anchored to kinetochores, centrosomes and mitochondria. Kinetochores are complexes of ~100 proteins which assemble at centromeres and serve as attachment points for spindle microtubules and regulatory hubs for mitotic checkpoint signalling [27] . To target Haloenzyme to kinetochores, we fused it to the kinetochore protein Nuf2, which localizes to the outer kinetochore, proximal to the microtubule binding site [30] . Centrosomes are protein-based organelles that are the primary microtubule organizing centers of animal cells. Centrosome replication and positioning are tightly regulated and linked to polarized cell division and cancer [31] , [32] , [33] . We used the centrosome targeting domain from AKAP9 (ref. 34 ) to localize Haloenzyme to centrosomes. Centromeres, kinetochores and centrosomes are not membrane-bound organelles. As a representative membrane-bound organelle, we chose mitochondria, which are involved in oxidative metabolism and apoptotic signalling, among many other critical cellular pathways. We targeted Haloenzyme to the cytosolic face of the mitochondrial outer membrane using the C-terminal domain of the Listeria monocytogenes ActA protein [35] . All three of these Haloenzyme–GFP-anchor constructs localized properly, and we successfully induced recruitment of mCherry–eDHFR to individual structures in all cases using short pulses (10–100 ms) of 405 nm laser illumination ( Fig. 6 ). Whole-cell activation of mitochondrial-targeted cTMP-Htag resulted in a dramatic depletion of free mCherry–eDHFR in the cytoplasm ( Supplementary Fig. 17 ). This result suggests that this system could be used for protein inactivation in a manner similar to rapamycin-induced re-routing [36] , with the added potential for spatial control (on the level of individual cells). Together, these results show that cTMP-Htag functions robustly at a membrane-bound organelle (mitochondria) and at three diverse non-membranous structures, including a DNA binding protein (CENPB) and two proteins which are localized entirely through protein–protein interactions (Nuf2 and AKAP9). The ability to selectively recruit a protein to an individual kinetochore within a pair of sister kinetochores separated by ~1 μm ( Fig. 6c ) highlights the power of this system for spatially precise manipulation of protein localization. 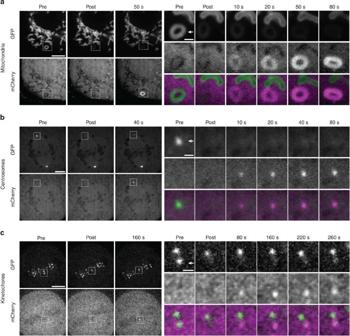Figure 6: Dimerization at individual mitochondria, centrosomes and kinetochores. Cells expressing mCherry–eDHFR and Haloenzyme–GFP-anchor domain fusion proteins specific for (a) mitochondria (ActA), (b) centrosomes (AKAP9) or (c) kinetochores (Nuf2) were incubated with 20 μM cTMP-Htag for 1 h, then washed before imaging. Cells were imaged before and after targeted laser illumination, as indicated. Individual structures in these cells (indicated by arrowheads in insets) were targeted with a 10–100 ms pulse from a 405 nm laser immediately before the ‘post’ image. Insets show boxed regions in GFP (top row) and mCherry (middle row) and colour-merge (bottom row) from indicated time points. GFP is locally photobleached by the 405 nm uncaging pulse. Gaussian smoothing with a radius of 1 pixel was applied to mCherry images inc. Scale bars, 5 or 1 μm in insets. Figure 6: Dimerization at individual mitochondria, centrosomes and kinetochores. Cells expressing mCherry–eDHFR and Haloenzyme–GFP-anchor domain fusion proteins specific for ( a ) mitochondria (ActA), ( b ) centrosomes (AKAP9) or ( c ) kinetochores (Nuf2) were incubated with 20 μM cTMP-Htag for 1 h, then washed before imaging. Cells were imaged before and after targeted laser illumination, as indicated. Individual structures in these cells (indicated by arrowheads in insets) were targeted with a 10–100 ms pulse from a 405 nm laser immediately before the ‘post’ image. Insets show boxed regions in GFP (top row) and mCherry (middle row) and colour-merge (bottom row) from indicated time points. GFP is locally photobleached by the 405 nm uncaging pulse. Gaussian smoothing with a radius of 1 pixel was applied to mCherry images in c . Scale bars, 5 or 1 μm in insets. Full size image We present a new strategy for controlling protein localization with light using a modular photocaged dimerizer covalently pre-localized to an anchoring protein. This technique should be readily and widely applicable at a variety of cellular locations to address a range of biological questions. We demonstrate localized light-induced protein recruitment to three structures (that is, centrosomes, centromeres and kinetochores) that have not been reported with any other published system, as well as mitochondria, a representative membrane-bound organelle that has been previously targeted [8] . Possible applications for cTMP-Htag include recruitment of microtubule associated proteins (such as motors) to one of the two centrosomes in a mitotic spindle [37] , chromatin remodelling factors to individual centromeres or mitotic checkpoint signalling proteins to individual kinetochores [38] , [39] . There is precedent for similar experiments using chemically induced dimerization or constitutive tethering to operator arrays, but these lacked either spatial or temporal control. The ability to manipulate protein localization at individual cellular structures using cTMP-Htag will enable comparisons between experimentally perturbed and unperturbed structures within single cells, or the introduction of imbalances between naturally paired structures such as kinetochores and spindle poles. Each of the published systems for light-inducible dimerization has a particular set of strengths and weaknesses, and none has emerged as optimal for all the applications. One fundamental difference between cTMP-Htag and the natural light-sensitive protein systems is that photochemical uncaging is irreversible, whereas most light-sensitive dimerization proteins will relax to a non-dimerizing state in the dark. Irreversibility may be an advantage or disadvantage, depending on experimental context, and cTMP-Htag dimerization can be reversed by addition of free TMP, albeit without spatial control. Identifying the best dimerization system for a given experiment will likely require empirical comparison. One strength of this system is its modular design, in which each function of the molecule is devolved to a specialized, independent chemical component. Modularity also allows for future development of dimerizers with different properties. Alternative photocages could be used to allow uncaging at longer wavelengths, or the protein-binding ligands could be replaced to allow the use of a different receptor. For example, a completely orthogonal dimerizer could be designed by replacing the Halotag ligand with a SNAP-tag ligand [13] , TMP with dexamethasone [18] and NVOC with a redshifted coumarin-based photocage [23] , which would allow for two different proteins of interest to be selectively recruited using different wavelengths of light. An expanding toolkit for light-induced protein dimerization will enable an exciting new era of experimental cell biology, in which researchers can optically control protein localization and interactions. Dimerizer synthesis and characterization 1 and 2 were synthesized via a convergent scheme ( Supplementary Fig. 1 ). Amine-functionalized TMP and carboxylic acid-functionalized Haloligand intermediates were prepared following literature precedent [40] , [41] , [42] . The functionalized TMP intermediate was photocaged in a single step using commercially available NVOC (Sigma-Aldrich) [43] . In the final, convergent step, the Haloligand module was coupled to either photocaged TMP or non-caged TMP via standard amide coupling conditions. Synthesis, purification and characterization of all products are detailed in Supplementary Figs 2–15 and Supplementary Methods . Ultraviolet–visible absorption spectrophotometry in Fig. 2 was performed on a JASCO V-650 spectrophotometer with a PAC-743R multichannel Peltier using quartz cells with a 1 cm cell path length. Cell culture and transfection All experiments were performed with HeLa cells [44] (obtained from E.V. Makayev, Nanyang Technological University, Singapore) either stably or transiently transfected with a plasmid for bicistronic expression of mCherry–eDHFR and indicated Haloenzyme constructs (see below). CENPB and mitochondria experiments were performed with stable cell lines; centrosome and kinetochore experiments were performed by transient transfection. Stable cell lines were created by recombinase-mediated cassette exchange using the HILO recombinase-mediated cassette exchange system [44] (obtained from E.V. Makeyev, Nanyang Technological University, Singapore). Briefly: a monoclonal acceptor cell line with LoxP and Lox2272 recombination sites at a single chromosomal locus was cotransfected with a donor plasmid containing a transgenic cassette flanked by LoxP and Lox2272 sites and a second plasmid expressing Cre recombinase, followed by selection for a marker in the donor cassette. Cells were cultured in growth medium (Dulbecco’s Modified Eagle’s medium with 10% FBS and penicillin–streptomycin) at 37 °C in a humidified atmosphere with 5% CO 2 . Cells at ~60% confluency in a single well of a 6-well plate were transfected with 1 μg of donor plasmid+10 ng of Cre plasmid pEM784 (see below for plasmid details) using 3 μl of Fugene 6 (Promega). Two days after transfection, 1 μg ml −1 puromycin was added to the growth medium for the selection of stable cell lines. Transient transfections were performed as above using 3 μl of Fugene 6 and 1 μg of plasmid DNA, 40 h before experiment. Dimerizer treatment cTMP-Htag ( 1 ) was dissolved in dimethyl sulphoxide at 10 mM and stored in amber plastic microcentrifuge tubes at −80 °C, then diluted in medium to a final working concentration of 20 μM (except as indicated in Fig. 3 ). Care was taken to minimize incidental exposure of cTMP-Htag or treated cells to light before the experiment. We found that working quickly in low levels of normal room lighting did not cause any detectable premature uncaging. The low levels of white light necessary for differential interference contrast microscopy also did not cause any detectable cTMP-Htag uncaging. TMP-Htag ( 2 ) and Halo-OreGrn were dissolved in dimethyl sulphoxide at 10 mM and 100 μM, respectively, and stored at −80 °C. Plasmids and primers pEM784, expressing nuclear-localized Cre recombinase and the donor cassette plasmid pEM705 were obtained from E.V. Makeyev [44] . All the dimerization protein expression plasmids used for this study were derived from pEM705, which contains a CAG promoter and a viral Internal Ribosome Entry Sequence (IRES) for constitutive bicistronic cDNA expression in mammalian cells. For this study mCherry–eDHFR was cloned downstream of the IRES, and the Haloenzyme constructs were cloned upstream of the IRES. For centromere experiments in Figs 4 and 5 , and Supplementary Fig. 16 , the full sequence of human CENPB was fused to the N terminus of GFP-Haloenzyme to produce CENPB–GFP–Haloenzyme. For centromere experiments in Fig. 3 , the DNA binding domain (DBD) comprising the first 167 amino acids of human CENPB was fused to the N terminus of Haloenzyme to produce CENPB DBD –Haloenzyme. For mitochondrial targeting in Fig. 6a and Supplementary Fig. 17 , the mitochondrial outer membrane targeting domain comprising the C-terminal 47 amino acids of the Listeria monocytogenes ActA gene was fused to the C terminus of Haloenzyme–GFP. For centrosome targeting in Fig. 6b , the PACT (Pericentrin and AKAP Centrosome Targeting) domain of AKAP9 (residues 3642–3807) was fused to the C terminus of Haloenzyme–GFP. For kinetochore targeting in Fig. 6c , the full sequence of the human outer kinetochore protein Nuf2 was fused to the C terminus of Haloenzyme–GFP. All primers used for cloning were obtained from Integrated DNA Technologies. The following primers were used: mCherry forward 5′-acgatgataatatggtgagcaagggcgaggagg-3′ and reverse 5′-tctagactccaggccggccttatacagctcg-3′; eDHFR forward 5′-ggcctggagtctagaatcagtctgattgcggc-3′ and reverse 5′-cgcctcgagcgcttaattaaagatcctcttctgagatgagtttttgttcc-3′; CENPB DBD forward 5′-ccggcgcgccaccggtcaccatgggccccaagagg-3′ and reverse 5′-ttctgcaccacgcgtcccgccactgccctccgag-3′; C-terminal Haloenzyme forward 5′-acgcgtggtgcagaaatcggtactggctttccattcg-3′ and reverse 5′-taggctgcagaccggctagccggaaatctcgagcgtcgac-3′; full-length CENPB-GFP forward 5′-ccggcgcgccaccggtcaccatgggccccaagaggc-3′ and reverse 5′-tttctgcaccacgcgtttcaccacccttgtacagctcgtc-3′; N-terminal Haloenzyme forward 5′-atcaccctgcagtacggcgcgccaccatggcagaaatcggtactggctttcc-3′ and reverse 5′-atatcaagcttatcgtcatccggaaatctcgagcgtcgac-3′; GFP forward 5′-gctcgagatttccggttacgtagccaccatggtgagcaagggc-3′ and reverse 5′-cttatcgtcatccggattcaccacccttgtacagctcgtc-3′; ActA forward 5′-gggtggtgaatccggtgatgcatcgggaagtggaagtggatctcgagc-3′ and reverse 5′-cttatcgtcatccggagatcagttatctagatccggtggatcc-3′; AKAP9 forward 5′-gggtggtgaatccggtgatgcatcgtatcgattgctagccaacattgaagcc-3′ and reverse 5′-cttatcgtcatccggatgcaccttgattcagtccaaagccatctc-3′; Nuf2 forward 5′-gggtggtgaatccggtgatgcatcgcgagctcaagcttcgaattcaggc-3′ and reverse 5′-cttatcgtcatccggacattttgaacatcttcctcttcagttcagc-3′. Image acquisition and photoactivation For live imaging, cells were plated on 22 × 22 mm glass coverslips (no. 1.5; Fisher Scientific) coated with poly-D-lysine (Sigma-Aldrich) or 4-chamber CELLview #1.5 glass coverslip 35 mm dishes (Greiner Bio-One). Coverslips were mounted in magnetic chambers (Chamlide CM-S22-1, LCI). During imaging, cells were maintained in L-15 medium without phenol red (Invitrogen) supplemented with 10% FBS and penicillin/streptomycin. Temperature was maintained at ~35 °C using an environmental chamber (Incubator BL; PeCon GmbH). All images were acquired with a spinning disk confocal microscope (DM4000; Leica) with a × 100 1.4 NA objective, an XY Piezo-Z stage (Applied Scientific Instrumentation), a spinning disk (Yokogawa), an electron multiplier charge-coupled device camera (ImageEM; Hamamatsu Photonics), and a laser merge module equipped with 488- and 593-nm lasers (LMM5; Spectral Applied Research) controlled by MetaMorph software (Molecular Devices). Images in Figs 4 , 5 , 6 and Supplementary Figs 16 and 17 are single confocal sections, images in Fig. 3 are maximum-intensity projections of five confocal sections, 1 μm spacing. For whole-cell ultraviolet exposure experiments in Figs 4a and 5a , and Supplementary Figs 16a and 17 , light from a mercury arc lamp (Osram HXP R 120W/45c Vis) was filtered through a 387/11 nm bandpass filter (Semrock part #FF01-387/11 as a component in a 4',6-diamidino-2-phenylindole filter cube) and focused through the objective. Targeted laser experiments in Figs 4c and 6 used an iLas2 illuminator system (Roper Scientific), equipped with a 405 nm laser (CrystaLaser LC model # DL405-050-O) with a measured output of 27 mW after fibre coupling, controlled using the iLas2 software module within Metamorph. Individual centromeres, mitochondria, centrosomes and kinetochores were photoactivated by defining rectangular regions of interest (2–6 μm 2 , depending on the individual structure) and rasterized 10 times with the laser at 15% power. Other standard commercial imaging systems, such as a scanning confocal microscope, could also be used for these experiments. Image processing All image processing and analysis was performed using ImageJ [45] . Image quantification in Figs 3 was performed on maximum-intensity Z-projections (five confocal sections, 1 μm spacing). Image quantification in Supplementary Fig. 17 was performed on single confocal sections. For mCherry–eDHFR recruitment quantification in Figs 4 and 5 , centromere regions were defined by thresholding the GFP channel using the MaxEntropy algorithm. Whole-cell regions were defined by thresholding the mCherry channel using the Huang algorithm. Average mCherry intensity values within the centromere and whole-cell regions were measured. Whole-cell average mCherry intensity was subtracted from centromere mCherry intensity for each time point. These values were normalized over the entire time course for each field, then normalized centromeric intensities were averaged over all the fields at each time point. For Halo-OreGrn staining quantification in Fig. 3 , centromere regions were defined in the green fluorescence channel using the MaxEntropy algorithm. Average background intensity was measured in several areas between cells and subtracted from the average centromeric green fluorescence values for each field. These background-subtracted values were then averaged over all the fields for each condition. How to cite this article : Ballister, E. R. et al. Localized light-induced protein dimerization in living cells using a photocaged dimerizer. Nat. Commun. 5:5475 doi: 10.1038/ncomms6475 (2014).